Photoredox cooperative N-heterocyclic carbene/palladium-catalysed alkylacylation of alkenes Three-component carboacylation of simple alkenes with readily available reagents is challenging. Transition metal-catalysed intermolecular carboacylation works for alkenes with strained ring or directing groups. Herein, we develop a photoredox cooperative N-heterocyclic carbene/Pd-catalysed alkylacylation of simple alkenes with aldehydes and unactivated alkyl halides to provide ketones in good yields. This multicomponent coupling reaction features a wide scope of alkenes, broad functional group compatibility and free of exogenous photosensitizer or external reductant. In addition, a series of chlorinated cyclopropanes with one or two vicinal quaternary carbons is obtained when chloroform or carbon tetrachloride is used as the alkyl halide. The reaction involves the alkyl radicals from halides and the ketyl radicals from aldehydes under photoredox cooperative N-heterocyclic carbene/Pd catalysis. Transition metal (TM)-catalyzed vicinal dicarbofunctionalization of alkenes is a powerful protocol for the construction of two C–C bonds to give value-added molecules from simple starting materials [1] , [2] , [3] , [4] . Particularly, the TM-catalyzed alkene carboacylation reactions provide easy access to ketones, which are key structural motifs in many natural products [5] , [6] . The intramolecular carboacylation under TM catalysis has been well established, including carboacylation with acylquinolines [7] , [8] , [9] , [10] , reactions of alkenes tethered with ring-strained cyclobutanones [11] , [12] , [13] , unstrained ketones [14] , and amides [15] , etc. However, the intermolecular TM-catalyzed carboacylation has been far less developed. The Rh-catalyzed intermolecular carboacylation of alkenes with the directing group was reported by Douglas in 2009 [16] . Later, the Pd- or Ni-catalyzed carboacylation of norbornene with amides or esters using triarylborane as the arylation reagent was developed [17] , [18] . The nickel-catalyzed carboayclation with acyl chloride and perfluoroalkyl iodide was recently reported by Chu et al. [19] . Apparently, the requirement of alkenes with a strained ring or directing group and the employment of perfluoroalkyl reagents limits the potential application of those reactions. N -Heterocyclic carbene (NHC) catalysis has evolved as a powerful tool for the construction of various organic molecules [20] , [21] , [22] , [23] , [24] . Recently, the NHC-catalyzed radical reactions provide possibility for chemical transformations (Fig. 1a ) [25] , [26] , [27] , [28] . In 2019, Ishii et al. disclosed the NHC-catalyzed radical decarboxylative coupling of aldehydes with N -hydroxyphthalimide (NHP) esters [29] , [30] . Laterly, pyridinium salts [31] , Togni reagents [32] , [33] , [34] , and activated perfluoroalkyl reagents [35] were used as the alkyl radical precursors for the NHC-catalyzed redox reactions. In addition, the generation of radical intermediates via photoredox has also been explored in NHC catalysis (Fig. 1b ) [36] , [37] , [38] , [39] , [40] . Our group reported the merging of NHC catalysis and photoredox catalysis for γ- and ε-alkylation with electron-deficient alkyl halides [41] . Scheidt [42] , [43] and Studer [44] developed the dual NHC and photoredox catalysis using benzyl Hantzsch esters or the Langlois reagents as alkyl radical precursor, respectively. However, compared to these active alkyl radical precursors, the utility of simple but unactivated alkyl halides remains underexplored due to their low reduction potential [45] . In the last decade, the combination of NHC with TM catalysis has made great progress to promote reaction otherwise impossible (Fig. 1c ) [46] . While most of the reactions involve the TM-allylic/propargyl intermediate [47] , [48] , [49] , [50] , [51] , [52] , [53] , [54] , [55] , the reaction of simple and less active alkene meets challenge [56] . Fig. 1: Redox NHC and cooperative NHC/TM catalysis. a Redox NHC-catalyzed radical reactions. b The merging of photoredox and NHC catalysis. c The combination of NHC with TM catalysis. d Our strategy: photoredox cooperative NHC/palladium-catalyzed alkylacylation of alkenes. TM transition metal, LG leaving group, X halide, SET single-electron transfer. Full size image Here, we develop a photoredox cooperative NHC/Pd-catalyzed alkylacylation of simple alkenes with aldehydes and unactivated alkyl halides (Fig. 1d ). This reaction involves the coupling of ketyl radical from aldydes [57] and alkyl radicals from halides [58] , [59] , [60] , [61] , delivering a range of ketones in good to high yields. 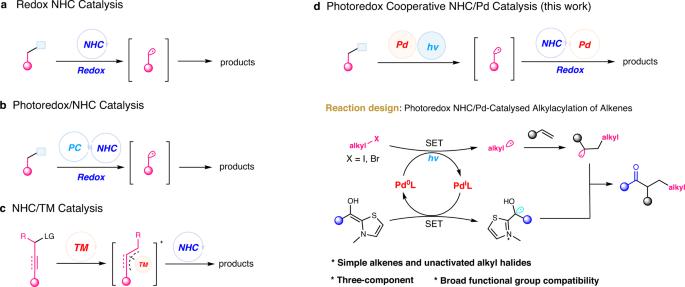Fig. 1: Redox NHC and cooperative NHC/TM catalysis. aRedox NHC-catalyzed radical reactions.bThe merging of photoredox and NHC catalysis.cThe combination of NHC with TM catalysis.dOur strategy: photoredox cooperative NHC/palladium-catalyzed alkylacylation of alkenes. TM transition metal, LG leaving group, X halide, SET single-electron transfer. Condition optimization of the alkylacylation Initially, the model alkylacylation of 2-vinylnaphthalene 1a with 2-pyridinecarboxaldehyde 2a and commercially available trimethyl(iodomethyl)silane 3a was explored under photoredox cooperative NHC/Pd catalysis (Table 1 ). We were happy to find the desired three-component coupling product 4 was isolated in 78% yield without Heck-type byproduct when the reaction was carried out in the presence of 10 mol% of Pd(OAc) 2 with t Bu-Xantphos L1 as the ligand, 20 mol% thioazolium preNHC N1 with Cs 2 CO 3 as the base and 20 mol% 4-methylpyridin-2-ol A1 as the additive [62] in 1,4-dioxane under blue LED irradiation (entry 1). Control experiments showed that the yield was somewhat decreased without additive or use of additive A2 instead of A1 (entries 2 and 3). The use of ligand Cy-Xantphos L2 , Xantphos, DPEphos or rac -BINAP instead of L1 resulted in trace product (entries 4–5). Using THF or toluene as the solvent showed no strong influence on this reaction (entry 6). Other palladium catalysts such as Pd(PPh 3 ) 2 Cl 2 , Pd(PPh 3 ) 4 and Pd 2 (dba) 3 were far less effective (entry 7). The screening of preNHC catalysts revealed that thioazolium preNHC N2 and N3 resulted in some loss of the yield (entry 8), while triazolium preNHC N4 did not work, possibly due to the shorter lifespan of the ketyl radical from triazolium NHC than thioazolium [57] (entry 9). Screening of bases showed that DBU and K 2 CO 3 performed much better than Na 2 CO 3 possibly due to its lower basicity (entries 10–11). Lowering the loading of preNHC N1 to 10 mol% resulted in decreased yield (entry 12). Finally, the reaction did not work in the absence of light, preNHC, Pd(OAc) 2 , or Ligand L1 (entry 13). Table 1 Condition optimization a Full size table Substrate scope With the optimized reaction conditions in hand, the generality of the photoredox cooperative NHC/palladium-catalyzed alkylacylation reaction was then investigated (Fig. 2 ). It was found that all styrenes with electron-rich and electron-deficient substituents at the para positions of the phenyl moiety are capable partners for this transformation, providing the desired ketones in moderate to good yields ( 5 – 16 ). Functional groups such as aldehyde, nitro, and alkynyl were also compatible ( 17 – 19 ). Both 1-vinylnaphthalene and styrenes with meta- or ortho- substituents worked well ( 20 – 24 ). Pentafluorostyrene and those with heteroaryl such as 2-pyridyl, 2-thienyl and 2-benzofuryl group were also amenable, affording the corresponding ketones in moderate to good yields ( 25 – 28 ). In addition, the reaction of 1-methyl-1-phenylethylene went smoothly to give ketone 29 with quaternary carbon in 71% yield. However, 1 H -indene (internal alkene), allylbenzene (aliphatic alkene), and butyl methacrylate (Michael acceptor) were unreactive under current conditions. Fig. 2: Substrate scope for alkylacylation of alkenes. Reaction conditions: 1 (0.20 mmol), 2 (0.40 mmol), 3 (0.3 mmol), Pd(OAc) 2 (10 mol%), L1 (12 mol%), N1 (20 mol%), A1 (20 mol%), Cs 2 CO 3 (150 mol%), 2.0 mL 1,4-dioxane, rt, blue LED (36 W) under N 2 ; X = I, unless otherwise noted. a X = Br; b 1 (0.40 mmol), 2 (0.20 mmol), and 3 (0.3 mmol) were used. Full size image The scope of aldehydes was then explored. Heteroaromatic aldehydes, such as furfural, thiazole-4-carboxaldehyde, 2-methylthiazole-4-carboxaldehyde, 2-pyridinecarboxaldehydes and 4-pyridinecarboxaldehyde, showed good reactivity under standard conditions ( 30 – 36 ). Benzaldehyde and those with para- and meta- substituents (R = 4-F, -Cl, -Br, -CF 3 , -CN and 3-Cl) all worked for the alkylacylation reaction, giving the corresponding α-aromatic ketones in good yields ( 37 – 43 ). It is noteworthy that the acidic hydroxyl group in salicyladehydes showed no harm to the reaction, giving the expected ketones 44 – 46 in good yields. Variation of the halides showed that all primary haloalkanes with less or more steric alkyl group reacted efficiently to furnish the coupling products 47 − 50 in good to high yields. Both secondary and tertiary haloalkanes worked well for the reaction, although two equivalent alkenes were employed to circumvent possible direct coupling of aldehydes with the more stable alkyl radicals ( 51 – 58 ). The additional chlorine in bromoalkanes or idoalkanes showed no negative effect for the reaction with exclusive chemical selectivity ( 59 – 61 ). The reaction of trifluorohaloalkanes, such as 1,1,1-trifluoro-2-iodoethane and 1,1,1-trifluoro-3-iodopropane, went smoothly to give the fluorinated ketones 62 – 63 in high yields. The benzylic radical worked as well as the alkyl ones, affording the corresponding ketone 64 in good yield. The additional ether or amine functional group in alkyl halides were tolerable ( 65 – 66 ). Furthermore, the α-haloesters, such as bromoacetate, 2-methyl-2-bromopropionate and difluorobromoacetate, were also suitable radical precursors for the reaction ( 67 – 69 ). Cyclopropanes are privileged structure motif in natural products and bioactive compounds and useful building blocks in organic synthesis [63] . It is interesting that cholorcyclopropyl ketone 70 was obtained in good yield with excellent diastereoselectivity when CHCl 3 was used as the radical precursor for the alkylacylation reaction (Fig. 3 ). It was proposed that the cyclopropyl ketone was formed from alkylacylation product 70a by an intramolecular S N 2 cyclization under basic condition. More examples of the cascade alkylacylation/cyclopropanation were then examined (Fig. 4 ). It was found that 2-naphthaldehyde and benzaldehydes substituted with 4-F, 4-Cl, and 4-CF 3 all worked well to give the desired cyclopropanes in good yields with good to excellent diastereoselectivities ( 70 – 74 ). In addition, when carbon tetrachloride was used, the corresponding challenging dichlorocyclopropanes with vicinal four-substituent 75 – 79 were afforded in moderate to good yields. Fig. 3: Synthesis of cholorcyclopropyl ketone 70. Alkylacylation using chloroform as alkyl halide gave chloorocyclopropyl ketone as the final product. Full size image Fig. 4: Cascade alkylacylation/cyclopropanation. Reaction conditions: 1m (0.20 mmol), 2 (0.40 mmol), 3w (2.0 mmol) or 3x (1.0 mmol), Pd(OAc) 2 (10 mol%), L1 (12 mol%), N1 (20 mol%), A1 (20 mol%), Cs 2 CO 3 (250 mol%), 2.0 mL 1,4-dioxane, rt, blue LED (36 W) under N 2 . Full size image The potential utility of the reaction was demonstrated by gram-scale experiment and further chemical transformations of the resulted ketone (Fig. 5 ). The α-aromatic ketone 5 was obtained in 1.20 g, 81% yield from the reaction of 5.0 mmol of styrene. Alcohol 80 was resulted in 86% yield with 15:1 dr when ketone 5 was reduced by sodium borohydride (reaction a). The addition of ethynyl Grignard reagent to ketone 5 gave the corresponding alcohol 81 in 99% yield with 25:1 dr (reaction b). The Wittig reaction of ketone 5 with methyl ylide gave the corresponding olefin 82 in 67% yield (reaction c). Fig. 5: Gram-scale synthesis and further chemical transformations. a NaBH 4 , MeOH, 0 o C to rt. b THF, 0 o C to rt. c THF, 0 o C to rt. Full size image Mechanistic studies A series of control experiments were carried out to investigate the possible mechanism of the photoredox cooperative NHC/Pd-catalyzed alkylacylation reaction (Fig. 6 ). It was found that there was no alkylacylation product 4 detected when TEMPO was added as radical scavenger, while the adduct 83 from the alkyl radical and TEMPO was detected by HRMS (Fig. 6a ). The radical clock experiment using (bromomethyl)cyclopropane gave ketone 84 with rearrangement of cyclopropylmethyl radical (Fig. 6b ). The reaction with 6-bromohex-1-ene gave the ketone 85a with the formation of cyclopentyl ring as the major product (Fig. 6c ). These results strongly support the involvement of the alkyl radical as the key intermediate for the reaction. The reaction of (1-(2-phenylcyclopropyl)vinyl)benzene gave ketone 86 with ring-opening of cyclopropane, which supports the involving of benzyl radical species. Fig. 6: Mechanistic study. a Radical trapping experiment with TEMPO (2,2,6,6-tetramethylpiperidinooxy). b Radical clock experiment with (bromomethyl)cyclopropane. c Radical probe experiment with 6-bromohex-1-ene. d Radical clock experiment with (1-(2-phenylcyclopropyl)vinyl)benzene. Full size image The UV−Visible absorption spectra of possible combination of the substrates and reagents were then measured (Fig. 7 ). It was found that there was no apparent absorption for the solution of alkene, benzaldehyde, alkyl iodide, N -heterocylic carbene, phosphine ligand with alkyl iodide [64] , or the Breslow intermediate (NHC + benzaldehyde) in range of visible light (>400 nm), while absorption was observed in the same level for Pd/ligand, Pd/ligand/NHC and the full reaction mixture under the standard conditions. These results suggested that palladium species worked as photocatalysts for the reaction (see Supplementary Fig. 1 in SI for more details). Fig. 7: UV–Visible absorption spectra. The UV–Vis absorption spectra of possible combinations of the substrates and reagents. Full size image Then light on/off experiments were conducted (Fig. 8 ). These results reveal that the blue light is integral in the whole reaction process and excluded the chain-reaction process. Fig. 8: Light on/off experiments. The yield of ketone 4 determined by GC-MS using dodecane as an internal standard. 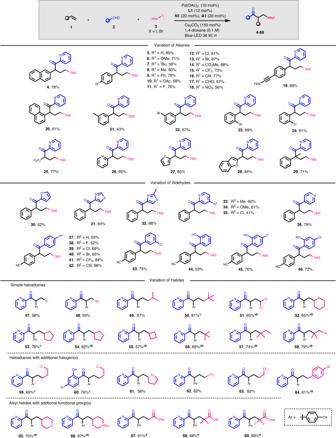Fig. 2: Substrate scope for alkylacylation of alkenes. Reaction conditions:1(0.20 mmol),2(0.40 mmol),3(0.3 mmol), Pd(OAc)2(10 mol%),L1(12 mol%),N1(20 mol%),A1(20 mol%), Cs2CO3(150 mol%), 2.0 mL 1,4-dioxane, rt, blue LED (36 W) under N2; X = I, unless otherwise noted.aX = Br;b1(0.40 mmol),2(0.20 mmol), and3(0.3 mmol) were used. Full size image Based on this information, the plausible catalytic cycle of the reaction was proposed as shown in Fig. 9 . The Pd 0 complex is excited under blue light irradiation, followed by a single-electron transfer (SET) between the photoexcited Pd 0 complex and alkyl halides 3 to give the Pd I complex and the alkyl radical species I . The addition of the alkyl radical to styrenes 1 produces radical species II . In the meantime, the Breslow intermediate III , generated from aldehydes 2 under NHC catalysis, is oxidized via an SET by Pd I complex to afford ketyl radical IV and Pd 0 complex. The radical-radical coupling between II and IV gives adduct V , which is fragmented to release the alkylacylation products and regenerate NHC catalyst. Fig. 9: Proposed catalytic cycle. The plausible mechanism for the photoredox cooperative NHC/Pd catalylsed alkylacylation of alkenes. Full size image In summary, we reported the photoredox cooperative NHC/Pd-catalyzed alkylacylation of alkenes with simple alkyl halides. This multicomponent coupling reaction used readily available starting materials with broad functional group compatibility. A wide range of aromatic aldehydes and simple alkyl halides directly coupled with styrenes, providing synthetically useful ketones in good to high yields. In addition, a series of chloro-cyclopropanes with quaternary carbon were obtained when chloroform or carbon tetracholoride was used as the alkyl radical precursor. This method does not require exogenous photosensitizers or external reductants. Mechanistic studies suggest the involvement of the alkyl radicals from halides and the ketyl radicals from aldehydes under photoredox cooperative NHC/Pd catalysis. Further mechanistic studies and reaction development are underway in our laboratory. 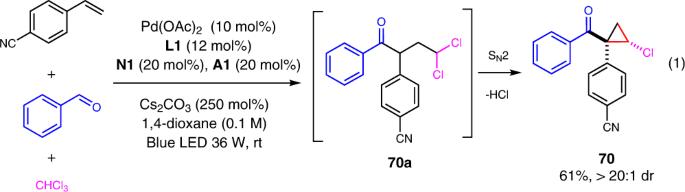Fig. 3: Synthesis of cholorcyclopropyl ketone 70. Alkylacylation using chloroform as alkyl halide gave chloorocyclopropyl ketone as the final product. General procedure for photoredox cooperative NHC/Pd-catalyzed alkylacylation of alkenes. A 4 mL vial equipped with a stir bar was charged with preNHC N1 (10.8 mg, 0.04 mmol), Pd(OAc)2 (4.5 mg, 0.02 mmol), ligand L1 (11.9 mg, 0.024 mmol) and 1.0 mL of 1,4-dioxane. After stirring for 30 min in glove box, to the solution was added Cs 2 CO 3 (97.8 mg, 0.3 mmol), additive A1 (4.4 mg, 0.04 mmol), alkenes 1 (0.2 mmol), aldehydes 2 (0.4 mmol), alkyl halides 3 (0.3 mmol), and 1.0 mL of 1,4-dioxane. The reaction mixture was removed from the glove box and stirred under 36 W blue LED lights at room temperature until the complete consumption of 1 (generally 48 h) by TLC analysis. The reaction mixture was filtered through a small pad of silica and eluted with EtOAc. 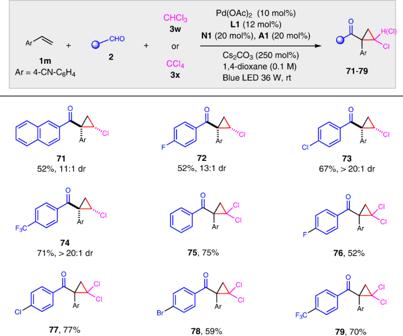Fig. 4: Cascade alkylacylation/cyclopropanation. Reaction conditions:1m(0.20 mmol),2(0.40 mmol),3w(2.0 mmol) or3x(1.0 mmol), Pd(OAc)2(10 mol%),L1(12 mol%),N1(20 mol%),A1(20 mol%), Cs2CO3(250 mol%), 2.0 mL 1,4-dioxane, rt, blue LED (36 W) under N2. 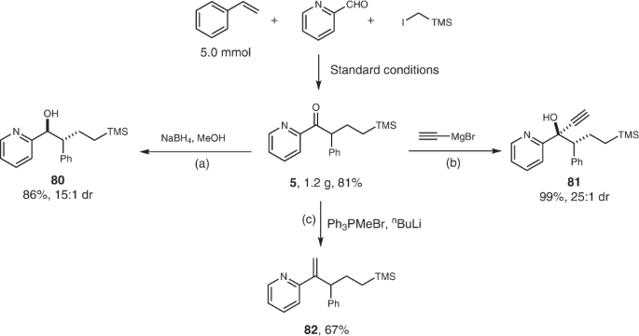Fig. 5: Gram-scale synthesis and further chemical transformations. aNaBH4, MeOH, 0oC to rt.bTHF, 0oC to rt.cTHF, 0oC to rt. 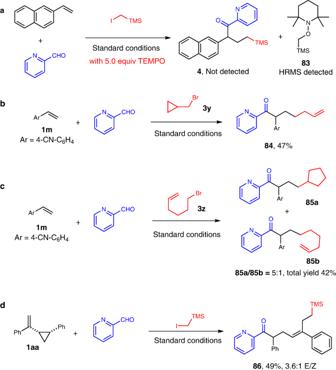Fig. 6: Mechanistic study. aRadical trapping experiment with TEMPO (2,2,6,6-tetramethylpiperidinooxy).bRadical clock experiment with (bromomethyl)cyclopropane.cRadical probe experiment with 6-bromohex-1-ene.dRadical clock experiment with (1-(2-phenylcyclopropyl)vinyl)benzene. 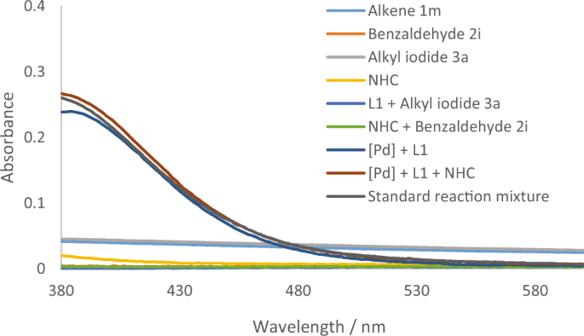Fig. 7: UV–Visible absorption spectra. The UV–Vis absorption spectra of possible combinations of the substrates and reagents. 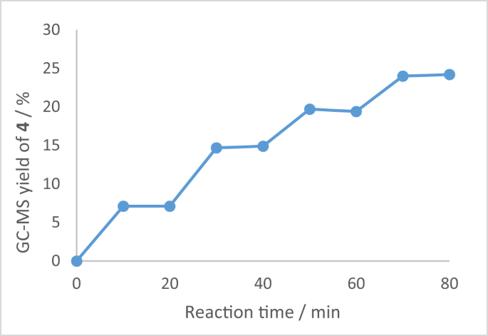Fig. 8: Light on/off experiments. The yield of ketone4determined by GC-MS using dodecane as an internal standard. 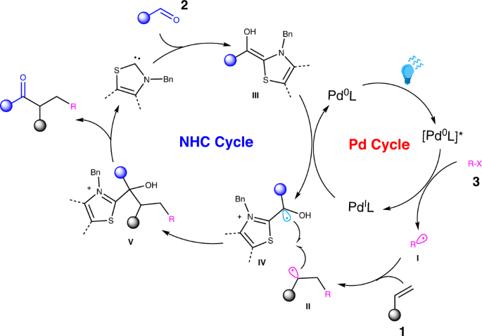Fig. 9: Proposed catalytic cycle. The plausible mechanism for the photoredox cooperative NHC/Pd catalylsed alkylacylation of alkenes. The solution was concentrated under reduced pressure, and purified by column chromatography on silica gel to afford the desired ketones (see SI for more details on experimentation).